Nearly 100% selective and visible-light-driven methane conversion to formaldehyde via. single-atom Cu and Wδ+ 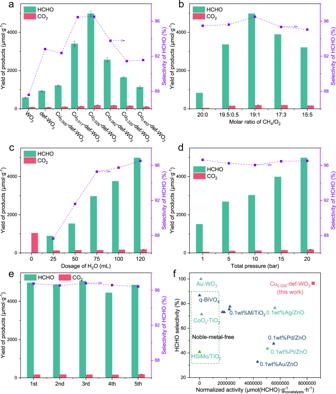Fig. 1: Selective CH4oxidation. aHCHO production over WO3, def-WO3and Cux-def-WO3photocatalysts in 2-h reaction. Optimisation ofbmolar ratio of CH4to O2,cH2O dosage anddtotal pressure of CH4and O2mixture on HCHO production over Cu0.029-def-WO3.eReusability of Cu0.029-def-WO3under five-cycle run.fComparison of CH4conversion to HCHO over Cu0.029-def-WO3and the typical reported photocatalysts10,18,19,20,77. Reaction conditions ina: 5 mg photocatalyst, 120 mL distilled H2O, 420 nm light irradiation and operated at 25oC. Reaction conditions inb,c,dare identical toaexcept varied O2pressure, H2O dosage and total pressure, respectively. Direct solar-driven methane (CH 4 ) reforming is highly desirable but challenging, particularly to achieve a value-added product with high selectivity. Here, we identify a synergistic ensemble effect of atomically dispersed copper (Cu) species and partially reduced tungsten (W δ+ ), stabilised over an oxygen-vacancy-rich WO 3 , which enables exceptional photocatalytic CH 4 conversion to formaldehyde (HCHO) under visible light, leading to nearly 100% selectivity, a very high yield of 4979.0 μmol·g −1 within 2 h, and the normalised mass activity of 8.5 × 10 6 μmol·g -1 Cu ·h −1 of HCHO at ambient temperature. In-situ EPR and XPS analyses indicate that the Cu species serve as the electron acceptor, promoting the photo-induced electron transfer from the conduction band to O 2 , generating reactive •OOH radicals. In parallel, the adjacent W δ+ species act as the hole acceptor and the preferred adsorption and activation site of H 2 O to produce hydroxyl radicals (•OH), and thus activate CH 4 to methyl radicals (•CH 3 ). The synergy of the adjacent dual active sites boosts the overall efficiency and selectivity of the conversion process. The rapid transition towards net-zero carbon (CO 2 ) emissions is an imperative undertaking by science and society to stave off potentially catastrophic climate change [1] . Hence, urgency arises: (1) to develop low-carbon transition pathways to turn traditional fossil resources into high-value-added chemicals, and (2) to displace traditional carbon-intensive manufacturing processes. Formaldehyde is an important high-volume industrial chemical with a market value of over 8 billion USD, expanding at a compound annual growth rate (CAGR) of 5.7%. It is widely used for household, commercial, aviation, medical and automotive products, and is a valuable precursor for melamine, urea-formaldehyde and phenolic resins, etc., due to its high reactivity and versatility [2] . It is also safely in use for the manufacture of vaccines, anti-infective drugs and hard-gel capsules. Currently, formaldehyde is produced by methanol oxidation-dehydrogenation using silver or metal-oxide catalysts at a high reactor temperature of over 500–600 °C, incurring both high CO 2 emission and energy penalties. On the other hand, with the continuous discovery of abundant methane (CH 4 ) resources, especially shale/natural gas, the direct CH 4 conversion into value-added chemicals such as methanol, formaldehyde and formic acid offers considerable economic and environmental benefits [3] , [4] , [5] , [6] , [7] . However, due to the high C–H bond dissociation energy (439 kJ·mol −1 ), CH 4 serves as the most stable and inert industrial feedstock among alkanes [8] , [9] , [10] , [11] , [12] , and its industrial utilisation through indirect steam-reforming and subsequently Fischer-Tropsch synthesis is usually energy-intensive due to the high operating temperature (700–1100 °C) [13] , [14] , [15] , [16] . Therefore, sustainable CH 4 utilisation under mild conditions is highly desirable. As a renewable technology, photocatalysis has shown unprecedented opportunities for overcoming thermodynamic barriers and achieving direct CH 4 conversion to various chemicals at ambient temperature. Recently, several efforts on direct photocatalytic CH 4 oxidation to methanol (CH 3 OH) and formaldehyde (HCHO) have been reported. High selectivity to CH 3 OH (>90%) and HCHO (100%) but with very moderate yields (350 μmol·g −1 ·h −1 of CH 3 OH and 300 μmol·g −1 ·h −1 of HCHO), have been achieved over optimised FeO x /TiO 2 and Au/WO 3 photocatalysts, respectively [17] , [18] . Noble-metal (Au, Ag, Pd, Pt) modified ZnO and TiO 2 performed acceptable yields of various oxygenates but with relatively low selectivity and mainly under UV/near UV irradiation (<80%) [17] , [18] , [19] , [20] , [21] , [22] , [23] . These advances encourage further investigations especially in the search for low-cost noble-metal-free photocatalysts with wide-spectrum response and simultaneous optimisation of activity and selectivity. Extending photoabsorption and enhancing charge separation generally improve photoactivity on various solar-driven reactions such as H 2 O splitting [24] , [25] , CO 2 reduction [26] , [27] , organic synthesis [28] , [29] and contaminant elimination [30] , [31] . However, such an approach is insufficient for CH 4 conversion due to its rather low electron and proton affinity. Moreover, another challenge for the CH 4 conversion into desirable oxygenates (i.e., CH 3 OH and HCHO) is that the targeted oxygenates are usually more reactive than CH 4 , which tend to be over-oxidised, leading to poor selectivity [23] , [32] . Hence, rationally regulating CH 4 reaction dynamics and promoting charge separation are equally significant to tune the overall photocatalytic performance. In industry, HCHO is solely produced from CH 3 OH oxidation and accounted for 30% consumption of CH 3 OH [33] . Multi-step production from CH 4 via steam reforming, Fischer-Tropsch synthesis and methanol conversion is energy-intensive and requires harsh conditions [33] , [34] . Nevertheless, one-step conversion from CH 4 to HCHO with high selectivity and yield is still lacking and no commercial catalyst is available even for high temperature. Hence, it is highly desirable to develop a suitable catalyst and/or co-catalyst as a promising alternative to promote photoabsorption, enhance charge separation and optimise selectivity under mild conditions [35] . The key to realise such direct conversion and selectivity depends on regulating the reactive oxygen species (ROS), enhancing the conversion of methane and promoting timely desorption of the desired products, whilst suppressing its mineralisation to CO 2 [18] . Suitable redox cocatalysts can be beneficial to charge transfer and promote the activation of the adsorbed O 2 and H 2 O to form reactive oxygen species such as superoxide (·O 2 - ), hydroperoxyl (·OOH) and hydroxyl (·OH) radicals. Introducing point defects in the photocatalyst may also modulate local electronic environment, facilitating reactant polarisation, chemical adsorption and hence electron/hole trapping to promote charge separation [36] , [37] . The integration of such dual reaction sites can simultaneously address the concerns on both charge separation and surface reaction dynamics [38] , [39] . Besides, a highly dispersed co-catalyst, especially single atoms or atomic clusters with a low co-ordination number, provides unique reaction sites for ready identification of the active local environment for CH 4 conversion [40] , [41] , [42] . Accordingly, it is of considerable benefit to develop highly dispersed noble-metal-free dual-site coordinated catalysts. Herein, tungsten oxide (WO 3 ) nanocrystals were used as the substrate due to its visible-light responsive property largely extending natural light utilisation. Atomic copper co-catalyst and W δ+ sites associated with oxygen vacancies (O v ) were hybridised to regulate synergistically charge transfer and surface reaction dynamics. Under 420 nm light irradiation, CH 4 was converted to HCHO with 96.5% selectivity and a maximum time yield of 12.4 μmol·h −1 . Computational simulations indicated that O v are essential to stabilise the single Cu atoms and induce the formation of adjacent W δ+ sites. Further mechanistic investigations proved that Cu species acted as the electron acceptors, while W δ+ species facilitated hole transfer and the preferred adsorption and activation of H 2 O to generate reactive hydroxyl radicals and then activated CH 4 . The ensemble co-ordination of the adjacent dual sites of single Cu atoms and W δ+ species thus resulted in the superior activity and selectivity of CH 4 conversion into HCHO at ambient temperature. Highly selective methane oxidation to formaldehyde by dioxygen CH 4 conversion reaction was conducted under 420 nm light irradiation with 120 mL distilled H 2 O, 1 bar O 2 and 19 bar CH 4 for 2 h at 25 °C. With no photocatalyst or light irradiation, no HCHO or other oxygenate products was detected, suggesting the critical role of photocatalyst and light irradiation. Over pristine WO 3 , relatively low yields of HCHO (579.5 μmol·g −1 ) and CO 2 (82.1 μmol·g −1 ) were produced (Fig. 1a ), which was mainly ascribed to the severe charge recombination over single-component nanocrystals compared with multicomponent photocatalysts that could facilitate charge separation and transfer [24] . The selectivity of HCHO was calculated to be 87.6%. To enhance photocatalytic CH 4 conversion efficiency, O v linked with W δ+ sites, as point defects, were introduced, due to the potential advantages of (i) improving light absorption through injection of sub-band gap or traps [43] , (ii) enhancing charge separation and transfer [36] , (iii) promoting chemical adsorption and activation of the symmetric molecule [37] . Defective WO 3– x (denoted def-WO 3 ) was prepared through temperature-programmed thermal reduction from pristine WO 3 in a hydrogen atmosphere (5 vol.% H 2 /Ar). Compared with the pristine counterpart, def-WO 3 showed 1.6 times higher HCHO production, being 933.2 μmol·g −1 . Moreover, only a trace amount of CO 2 by-products (72.2 μmol·g −1 ) was detected, indicating high selectivity of HCHO (92.8%) and significantly suppressed over-oxidation of CH 4 to CO 2 or CO. Fig. 1: Selective CH 4 oxidation. a HCHO production over WO 3 , def-WO 3 and Cu x -def-WO 3 photocatalysts in 2-h reaction. Optimisation of b molar ratio of CH 4 to O 2 , c H 2 O dosage and d total pressure of CH 4 and O 2 mixture on HCHO production over Cu 0.029 -def-WO 3 . e Reusability of Cu 0.029 -def-WO 3 under five-cycle run. f Comparison of CH 4 conversion to HCHO over Cu 0.029 -def-WO 3 and the typical reported photocatalysts [10] , [18] , [19] , [20] , [77] . Reaction conditions in a : 5 mg photocatalyst, 120 mL distilled H 2 O, 420 nm light irradiation and operated at 25 o C. Reaction conditions in b , c , d are identical to a except varied O 2 pressure, H 2 O dosage and total pressure, respectively. Full size image To further promote HCHO production, all period 4 transition metal elements, including Sc, Ti to Cu and Zn, were hybridised with the defective WO 3– x photocatalyst via. a highly reproducible impregnation method, along with subsequent thermal reduction. The as-prepared photocatalysts with different metal contents were denoted M x -def-WO 3 , where x % represented the actual mass percentage of the specific metal (M). The actual metal content was measured by inductively coupled plasma optical emission spectrometry (ICP-OES). Reaction evaluation under identical conditions (Fig. S1 ) suggested that Cu was the most suitable co-catalyst for HCHO production among these 3d metals. The intrinsic reason why Cu is the most effective among the selected 3d candidates lie not only in its ability to catalyse oxygen reduction reaction, but also its synergistic cooperation with the substrate to promote H 2 O oxidation so as to activate CH 4 as discussed below. The effect of copper content on HCHO production was then optimised, which exhibited a volcanic trend with increasing percentage of Cu, as shown in Fig. 1a . The highest HCHO yield was over Cu 0.029 -def-WO 3 (4979.0 μmol·g −1 ). Excessive Cu results in clustering, which may provide recombination centres for the charge carriers [44] . The dramatically enhanced activity is attributed to the increased availability of photo-generated charge carriers and efficient reactant activation as discussed below. Apart from the excellent HCHO production, a superior HCHO selectivity of 96.5% was also achieved. Moreover, a higher production rate means a higher HCHO concentration around the catalytic site, which may cause over-oxidation. However, no discernible level of CO 2 was detected, suggesting that the produced HCHO molecules could be desorbed from the surface of the catalyst in time to avoid deep oxidation. Effect of oxygen vacancy density on photocatalytic performance was also investigated by subtle control of the thermal reduction temperature with the same impregnated precursors. It was expected that a higher reduction temperature would lead to more O v via. oxygen extraction by H 2 . As shown in Fig. S2 , HCHO production reached the highest when it was prepared at 250 °C. Too high a temperature may result in the generation of deep trapping sites for charge recombination, while too low a temperature may not generate sufficient regulation of the structural defects. As shown in Fig. 1b–d , the reaction conditions, including the molar ratio of CH 4 to O 2 , H 2 O dosage and total pressure, were studied to optimise the HCHO production over Cu 0.029 -def-WO 3 . Initially, the effect of the molar ratio of CH 4 to O 2 was analysed, at a fixed pressure of 20 bar with varied CH 4 and O 2 dosages (Fig. 1b ). Without O 2 dosage, the HCHO conversion was 823.9 μmol·g −1 over Cu 0.029 -def-WO 3 , suggesting H 2 O could be the alternative oxygen source for HCHO. In the presence of a very small amount of molecular oxygen, HCHO production gradually increased with raising O 2 pressure. Further increasing O 2 while decreasing CH 4 pressure led to a reduction of HCHO production to 3210.2 μmol·g −1 at CH 4 /O 2 = 15/5. Such suppressed photoactivity would be primarily attributed to the reduced concentration of dissolved CH 4 . The optimal molar ratio of CH 4 to O 2 is 19:1, which is clearly higher than the stoichiometric ratio for the production of HCHO (CH 4 + O 2 → HCHO + H 2 O) and suggests a relatively large chemical gradient is needed to achieve an effective collision rate of the reactants at the catalytic local environment. Secondly, H 2 O dosage was studied under the optimised CH 4 /O 2 molar ratio (19/1). According to Raoult’s law, the molar ratio of the dissolved CH 4 /O 2 is fixed in water. By variation of the H 2 O dosage, the concentration of the photocatalyst varies, further influencing the light transmittance. As shown in Fig. 1c , the higher the H 2 O dosage, the higher the HCHO production. The trend is almost linear: With the gradual increase of H 2 O content from 25 to 120 mL, the HCHO production is enhanced from 890.5 μmol·g −1 to 4979.0 μmol·g −1 , corresponding to a concentration of HCHO from 178.1 μmol·L −1 to 207.5 μmol·L −1 , respectively (Fig. 1c ). The amount of oxidation of HCHO to CO 2 would be higher at a higher concentration of HCHO, as indeed observed here. The CO 2 production increases from 125.5 to 166.2 μmol·g −1 when water dosage is changed from 25 to 120 mL, or the concentration of HCHO varies from 178.1 to 207.5 μmol·L −1 . Interestingly, an improved selectivity to HCHO from 87.6% to 96.5% is also observed, suggesting that the change in CO 2 production does not affect the selectivity. Moreover, the HCHO production increases by ~4.6 folds from 890.5 to 4979.0 μmol·g −1 for the H 2 O dosage increase from 25 to 120 mL, respectively. Therefore, the dilution (or more water content) should preferentially promote the production and timely desorption of HCHO, rather than its oxidation on the surface of the photocatalyst. In other words, the increased HCHO production and selectivity can be attributed to the boosted light absorption and mass transfer of the products as a result of the higher amount of water used, at least under the range of H 2 O dosages considered here. More importantly, without H 2 O, a larger amount of CO 2 (1038.8 μmol·g −1 ) is detected, suggesting that H 2 O can suppress HCHO over-oxidation into CO 2 . This may be attributed to the solvation effect of H 2 O, promoting the desorption of oxygenate products [23] , [45] . Thirdly, the HCHO production was assessed over varying feeding pressure of CH 4 and O 2 under a constant molar ratio of 19 (Fig. 1d ). It reveals that HCHO production over Cu 0.029 -def-WO 3 responded almost linearly to the total feeding pressure. As mentioned above, this indicates that no side reaction occurred when increasing the dissolved CH 4 /O 2 at the constant ratio. The intrinsic HCHO product reached 1505.7 μmol·g −1 at ambient pressure. Finally, as shown in Fig. 1e , Cu 0.029 -def-WO 3 performed a relatively stable CH 4 conversion to HCHO, with no evident deactivation after five cycles, which confirms the stability of Cu 0.029 -def-WO 3 as a desirable photocatalyst. Meanwhile, the XRD (Fig. S3 ) and XPS spectra (Fig. S4 ) comparison of the freshly prepared Cu 0.029 -def-WO 3 and the one after 5 cycles exhibited no discernible difference. Meanwhile, copper was not detected in the filtered reactant by ICP-OES, which further suggests the stable topology of Cu 0.029 -def-WO 3 . The normalised mass activity was calculated using the formula ( \({{{{{\rm{Normalized\; activity}}}}}}=\,\frac{{{{{{\rm{n}}}}}}}{{{{{{\rm{m}}}}}}*{{{{{\rm{t}}}}}}}\) ), where n , m and t represent the molar production of HCHO (μmol), the mass of Cu co-catalyst (g) and reaction time (h), respectively. Comparison between the Cu 0.029 -def-WO 3 photocatalyst and typically reported photocatalysts for CH 4 conversion to HCHO is shown in Fig. 1f . Most of the photocatalysts show relatively low normalized activity for HCHO production. Some noble-metal-modified ZnO and TiO 2 photocatalysts under full-arc irradiation exhibit a higher normalized activity between 1.8 × 10 6 to 5.5 × 10 6 μmol (HCHO) ·g −1 (cocatalyst) ·h −1 , but the selectivity for HCHO is lower than 80% [19] . Regarding the selectivity, the best-performed Au-WO 3 catalyst presents a 100% HCHO selectivity but more than serval order of magnitudes lower normalized activity than our work [18] . Comparatively, the present noble-metal-free Cu 0.029 -def-WO 3 photocatalyst shows much superior photocatalytic activity with nearly 100% HCHO selectivity and a normalized activity as high as 8.5 × 10 6 μmol (HCHO) ·g −1 (cocatalyst) ·h −1 (with an apparent quantum yield of 1.14%) under 420 nm irradiation. Observation of active sites In order to clarify the mechanism of the high performance, we compared three samples (WO 3 , def-WO 3 and Cu 0.029 -def-WO 3 ), all of which show a typical and well-crystallised monoclinic WO 3 crystal structure (PDF#43-1035) as noted in the X-ray diffraction patterns (XRD) (Fig. S5 ). The incorporation of copper species through high-temperature reduction did not change the XRD patterns, indicating the stable topology of the WO 3 nanocrystal. In addition, there are no extra copper-associated diffraction peaks, due to its high dispersion and/or low loading. Raman spectra (Fig. 2a ) further support the WO 3 crystalline structure according to the typical WO 3 peaks observed at 130.8, 270.4, 713.2 and 804.2 cm −1 , which are contributed by lattice vibration, δ(O-W-O) deformation vibration and stretching ν(O-W-O) mode of the bridging oxygen of WO 3 , respectively [46] . Fig. 2: Structural characterisation. a Raman spectra and b high-resolution W 4f XPS spectra of WO 3 , def-WO 3 and Cu 0.029 -def-WO 3 . c HRTEM and d aberration corrected HAADF-STEM images of Cu 0.029 -def-WO 3 . e x – y line scan curve measured along the yellow rectangle region marked in d . f The optimised configuration of the atomic Cu at A site of def-WO 3 over the (002) surface in the top view. Full size image High-resolution X-ray Photoelectron Spectroscopy (XPS) was conducted to examine the chemical structure of the defective surface of the photocatalyst. As shown in Fig. 2b , the two deconvolution peaks from the W 4f XPS spectra at 35.65 and 34.56 eV are observed for the pristine WO 3 and attributed to W 6+ and W 5+ species, respectively. The minor amount of W 5+ species (3.4%) could be ascribed to the low concentration of the intrinsic defects in the nanocrystal [47] . For the def-WO 3 , the level of the W 5+ species increased to 14.4%, over 4 times higher than that of the counterpart, suggesting the successful introduction of O v linked with the W 5+ species. High-resolution O 1s XPS spectra (Fig. S6 ) provides further evidence of the successful introduction of O v , where the peak at 531.77 eV can be deconvoluted and ascribed to the O v [48] . The other two peaks centred at 530.32 and 532.88 eV can be assigned to the crystalline oxygen (W-O) and adsorbed moisture, respectively [49] . Accordingly, the results indicate that the hydrogen reduction is effective to introduce surface O v species, which regulate the local electronic environment and generate W δ+ sites therein [50] , [51] , [52] . Similar to those in the def-WO 3 , the percentages of W 5+ and O v species of the Cu 0.029 -def-WO 3 are 15.0% and 8.83%, respectively. This indicates that the O v are preserved after the Cu loading. Besides XPS spectra, O v are also confirmed through TEM images, EPR and UV-DRS as discusses later. The transmission electron microscopy (TEM) images of the pristine WO 3 and the def-WO 3 are shown in Fig. S7a , b and S8 , respectively. The former is characterised by a well-crystallised nanocrystal structure with smooth surfaces. High-resolution transmission electron microscopy (HRTEM) is accordance with the XPS analysis. Such defects in the subsurface are reported to result in electron delocalisation and benefit the stabilisation of reaction intermediates [53] , [54] , [55] . The crystalline d-spacings of 0.395 and 0.312 nm in Fig. 2c can be ascribed to (002) and (−112) facets of the WO 3 nanocrystal, respectively, indicating the primary structure of WO 3 is retained, consistent with the XRD observation. The unsaturated sites of the amorphous/defective layer should promote chemical adsorption and activation of the reactants [43] . Aberration corrected high-angle annular dark field scanning transmission electron microscopy (HAADF-STEM) images (Fig. 2d ) were captured to further investigate the dispersion of the copper species. Irregular tungsten atoms that present on the edge of the nanocrystal further support the existence of O v -induced W δ+ sites on the Cu 0.029 -def-WO 3 . Besides, it is also shown that W atoms distributed in the regular array, while some additional and smaller dots are clearly observed among the regular array, which may be assigned to Cu atoms. Cu K-edge X-ray absorption near edge structure (XANES) spectra of Cu 0.029 -def-WO 3 with Cu-foil and CuO references were then measured to further study the structural microenvironment of the Cu atoms (Fig. S10 ). Fourier transforms of the Cu K-edge (Fig. 3a ) exhibit only a predominant peak at ca. 1.51 Å for Cu 0.029 -def-WO 3 , which can be ascribed to the first shell of the Cu–O bond with reference to the CuO sample (Fig. S11 and Table S1 ). In parallel, no peaks corresponding to Cu-O-Cu and Cu-Cu at 2.47 Å and 2.23 Å were detected, confirming that the atomically dispersed Cu sites exist in the Cu 0.029 -def-WO 3 and are coordinated with oxygen. Fig. 3: Structural identification and photo-physical properties. a Fourier transforms of EXAFS of the Cu K-edge of Cu 0.029 -def-WO 3 , CuO and Cu-foil. Low-temperature in situ solid-state EPR spectra of b def-WO 3 and c Cu 0.029 -def-WO 3 under 420 nm irradiation for different time. d Steady-state PL spectra of WO 3 , def-WO 3 and Cu 0.029 -def-WO 3 . Full size image The x – y elemental line scan (Fig. 2e ) along with the yellow rectangle of Fig. 2d clearly shows the atomic dispersion of Cu in the oxide lattice. The distance between adjacent W and Cu atoms was measured as 0.201 nm along [001] crystalline direction of the (002) plane, which is consistent with the following density functional theory (DFT) calculation results that the O v is energetically favourable to host a single atomic Cu dopant (Fig. 2f and Fig. S12 ), where the direct line distance between the nearest W and Cu atoms is 0.434 nm. When projected normal to the [001] direction along the (002) plane, it is 0.218 nm, close to the experimental observation. Thus, the pristine (002) surface model was built based on the monoclinic WO 3 bulk structure, shown in Fig. S13a, b . The bottom two layers were fixed, while all other atoms were fully relaxed until the energy and force criteria were reached. The distance of the (002) surface is 3.91 Å, close to the experimentally measured value in this study (3.95 Å). The oxygen vacancy was created by the removal of a single oxygen atom on the top surface. After relaxation, the distance of the nearest W atom stretched to 4.34 Å (Fig. S14a ), compared to 3.85 Å in the pristine case. This open-site gives the energetically most favourable host position for an atomic Cu. Three possible adsorption sites were comparatively investigated, as shown in Fig. S14b–d , denoted as Site A, B and C, respectively. The optimised configurations are shown in Fig. 2f . The adsorption energy was calculated based on: 
    E_ad=E_total-E_O_v-E_Cu
 (1) where the \({E}_{{{{{{{\mathrm{total}}}}}}}}\) , \({E}_{{O}_{v}}\) and \({E}_{{{{{{{\mathrm{Cu}}}}}}}}\) are the energy of the whole system, that of the system with a single O vacancy on the WO 3 (002) surface and the chemical energy of copper, respectively. The results are listed in Table S2 . Both the A and the B sites are energetically favoured, but the A site is the most stable. The Bader charge analysis was carried out to evaluate the charge changes, and the results are listed in Table S3 . For the def-WO 3 , the Bader partial potential of the W atom decreases from −2.59e for the 2nd nearest to −2.34e for the nearest, suggesting a lowering of the valence of the nearest W δ+ ( δ < 6), induced by the oxygen vacancy. Such reduced oxidation states of W around the defect were also the case for the Cu-def-WO 3 , which strongly proves the existence of the W δ+ species at the active site. By accommodating the Cu in the A site (the most stable structure, also consistent with the HAADF-STEM images), the oxidation states of W decreased by 13% from −2.52e to −2.19e. This lends further benefit to W and Cu as the dual active sites for water and oxygen adsorption, respectively, as discussed later. Mechanistic investigation UV–Vis diffraction spectra (UV-DRS) (Fig. S15 ) show similar photoabsorption characteristics among WO 3 , def-WO 3 and Cu 0.029 -def-WO 3 , suggesting that photoabsorption is not the dominant factor influencing the photocatalysis herein. The absorption boundary at 426 nm determines the visible-light responsive properties of the as-prepared photocatalysts. Bandgap energies calculated by the Tauc plots (Fig. S16 ) are 2.91, 2.88 and 2.88 eV for WO 3 , def-WO 3 and Cu 0.029 -def-WO 3 , respectively. Additionally, Mott-Schottky plots (Fig. S17 ) were measured to establish the flat band position. Positive slopes of the Cu 0.029 -def-WO 3 photocatalyst indicate the n-type characteristics of WO 3 , for which the flat band always lies 0.1 V below the conduction band (CB) [56] . Thus, CB and valence band (VB) positions of the Cu 0.029 -def-WO 3 vs. NHE (pH = 0) are established as −0.10 and 2.78 V, respectively [57] , [58] . Therefore, the potentials of VB and CB positions are sufficient to drive O 2 reduction (−0.05 V vs. NHE) and H 2 O oxidation (2.38 V vs. NHE) to generate reactive species, such as ·OOH and ·OH radicals, respectively [59] , [60] . Electron paramagnetic resonance (EPR) is a highly sensitive tool for the study of the paramagnetic transition of metal ions and the oxygen vacancies due to unbalanced electron spins [61] . As shown in Fig. S18 , no evident EPR signal was detected for WO 3 , suggesting its pristine topology with no unpaired electrons. After the thermal reduction in hydrogen, the def-WO 3 exhibited a single Lorentzian EPR signal at g = 2.002, which can be assigned to an oxygen defective structure [49] . In the case of the Cu 0.029 -def-WO 3 , a similar EPR signal at g = 2.002 was also observed, but weaker than that of the def-WO 3 , thus indicating that the introduced copper species are very likely on/around O v so reducing its EPR response [62] . Meanwhile, an additional hyperfine peak at g = 2.061 is observed, which is attributed to the hybridized Cu 2+ species [63] , [64] . The hyperfine structure of this peak provides further evidence of the high dispersion of the copper species. In situ light-irradiated EPR spectra of the def-WO 3 and the Cu 0.029 -def-WO 3 were then tested to probe further details of the charge transfer mechanism. For the def-WO 3 , a newly added EPR signal at g = 2.007 was observed under light irradiation (Fig. 3b ), which is likely due to the excited electrons at the conduction band of WO 3 . In parallel, the signal of O v at g = 2.002 gradually becomes stronger under light irradiation, suggesting O v facilitate the trapping of active electrons from the conduction band and an equilibrium is reached after 120 s. In contrast, no noticeable change at g = 2.007 and 2.002 (Fig. S19 ) was observed for the Cu 0.029 -def-WO 3 under identical conditions, suggesting that the photo-induced electrons at the conduction band of WO 3 and the O v could efficiently migrate to the Cu species. In addition, the constant intensity of the Lorentzian signal at g = 2.002 would suggest that the O v serve as the mediator for electron transfer from the conduction band to the Cu species in the Cu 0.029 -def-WO 3 . Accordingly, a hyperfine EPR signal at g = 2.056 (Fig. 3c ) was observed for the Cu 0.029 -def-WO 3 , which is ascribed to the Cu 2+ species as Cu + and Cu 0 are EPR-silent. Under continued light irradiation, the Cu 2+ signal gradually weakens, indicating a reduced content of the Cu 2+ species, implying that the Cu 2+ serves as the electron acceptor. In situ Cu 2p XPS spectra (Fig. S20 ) with and without light irradiation were obtained for further investigation of the role of the Cu species. In dark, the deconvoluted Cu 2p XPS results validate the coexistence of Cu 0 /Cu + (932.38 eV) and Cu 2+ (933.60 eV) for the Cu 0.029 -def-WO 3 , which corresponds to the composition of 66% Cu 0 /Cu + and 34% Cu 2+ , respectively. Under light irradiation, the concentration of Cu 2+ dramatically decreased to 19% while Cu 0 /Cu + increased to 81%, further confirming the active role of Cu 2+ as the electron acceptor. Steady-state and time-decay photoluminescence (PL) spectra (Fig. 3d and S21 ) were conducted to study the charge transfer dynamics. The strong PL peak of the pristine WO 3 is correlated with its severe charge recombination, as expected for the single component [24] . Comparatively, the def-WO 3 shows relatively weaker PL intensity than WO 3 , indicating an enhanced charge separation efficiency [65] , which should originate from the role of O v in the def-WO 3 as the electron trapping sites. In the case of the Cu 0.029 -def-WO 3 , PL intensity decreased further, being the lowest, among the different Cu-based photocatalysts, implying the most suppressed charge recombination case after the incorporation of the atomic Cu. Notably, different from the def-WO 3 , the O v in the Cu 0.029 -def-WO 3 contribute little to charge separation, as evidenced by the unchanged EPR intensity under light irradiation (Fig. S19 ), suggesting the highly dispersed Cu co-catalyst is more efficient than the O v in acting as the photo-induced electron acceptors. DFT simulations were then employed to show the charge density distribution of the conduction band minimum (Fig. 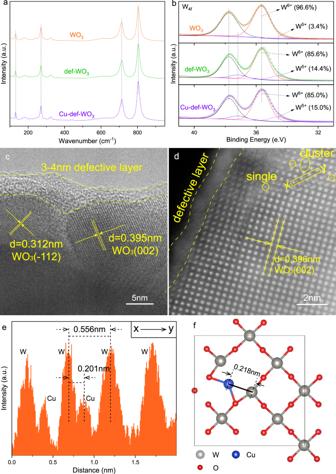Fig. 2: Structural characterisation. aRaman spectra andbhigh-resolution W4fXPS spectra of WO3, def-WO3and Cu0.029-def-WO3.cHRTEM anddaberration corrected HAADF-STEM images of Cu0.029-def-WO3.ex–yline scan curve measured along the yellow rectangle region marked ind.fThe optimised configuration of the atomic Cu at A site of def-WO3over the (002) surface in the top view. 4a ) and the valence band maximum (Fig. 4b ) of the Cu-def-WO 3 . The charges are found to significantly accumulate around the Cu and the O v region in the conduction band minimum (Fig. 4a ). From Bader charge analysis in Table S3 , the partial charge of the related O atom changes from 0.58e for the pristine WO 3 , to 1.06e for the def-WO 3 , and 0.98e for Cu-def-WO 3 . It confirms our speculations in EPR results. From the in situ EPR and XPS analyses, with further support from DFT simulations, it may be inferred that photo-excited electrons in the conduction band are firstly trapped by the O v , and then transferred to the Cu species to facilitate the formation of Cu + (Cu 2+ + e - → Cu + ), where Cu + would next act as the electron donor to activate the adsorbed O 2 on the surface (Cu + + O 2 → Cu 2+ + ·OO - ). Under reaction conditions in the presence of H 2 O, superoxide radicals (·OO - ) tend to react with a proton and form ·OOH radicals. In parallel, photo-induced holes locate around the hybridized O and W δ+ (Fig. 4b ). Fig. 4: Photo-chemical properties. a Conduction band minimum and b Valence band maximum charge distributions of Cu-def-WO 3 . The grey, red and blue balls represent W, O and Cu atoms, respectively. In situ EPR monitor of c ·OOH and d ·OH radicals trapped by DMPO over WO 3 , def-WO 3 and Cu 0.029 -def-WO 3 under light. e Time-dependent PL intensity of 7-hydroxycoumain from the reaction of coumarin and ·OH over WO 3 , def-WO 3 and Cu 0.029 -def-WO 3 . f GC-MS of the produced HCHO with isotopic labelled H 2 18 O or 18 O 2 in the presence of 19 bar CH 4 and 1 bar O 2 and 3 mL H 2 O over Cu 0.029 -def-WO 3 . Full size image Time-decay PL spectra (Fig. S22 ) were fitted by the two-exponential decay. All samples exhibit similar exponential emission properties. Compared with the WO 3 and the def-WO 3 , a much slower decayed emission of the Cu 0.029 -def-WO 3 demonstrates slower kinetics of the fluorescent decay and the suppressed charge recombination. The average PL lifetime of the Cu 0.029 -def-WO 3 was calculated to be 4.61 ns (Table S4 ), longer than that of the WO 3 (3.14 ns) and the def-WO 3 (3.27 ns), indicating that the Cu 0.029 -def-WO 3 most facilitates the charge carrier separation. Photocurrent responses were measured to evaluate further the charge separation dynamics. As shown in Fig. S23 , the def-WO 3 shows a photocurrent intensity of 12.2 μA·cm −2 , 1.9 times stronger than that of the pristine WO 3 (6.3 μA·cm −2 ), demonstrating the efficient transfer of photo-induced electrons to the defects. For Cu 0.029 -def-WO 3 , photocurrent density is further increased to 14.8 μA·cm −2 , about 1.2 times higher than that of the def-WO 3 , suggesting the role of the Cu species in promoting charge separation. Electrochemical impedance spectroscopy (EIS) plots (Fig. S24 ) show a much smaller radius of Cu 0.029 -def-WO 3 than those of def-WO 3 and WO 3 , indicating its smallest resistance for interfacial charge transfer. From the above analysis, it is clear that the charge recombination is greatly suppressed by suitable ensemble corporation of the O v -W δ+ sites and highly dispersed Cu-co-catalyst atoms, which result in efficient charge separation and transfer. Reactive oxygen species, including hydroperoxyl (·OOH) and hydroxyl radicals (·OH), were monitored with 5, 5-dimethyl-1-pyrroline N-oxide (DMPO) as the trapping agent by the detection of DMPO-OOH and DMPO-OH adducts, respectively. The intermediate of O 2 reduction was measured in methanol solution under light irradiation (Fig. 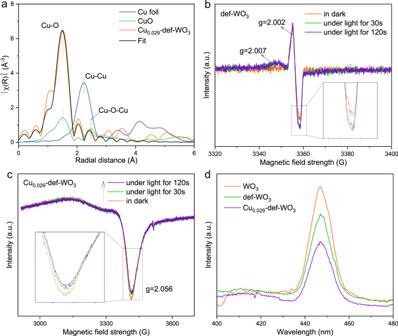Fig. 3: Structural identification and photo-physical properties. aFourier transforms of EXAFS of the Cu K-edge of Cu0.029-def-WO3, CuO and Cu-foil. Low-temperature in situ solid-state EPR spectra ofbdef-WO3andcCu0.029-def-WO3under 420 nm irradiation for different time.dSteady-state PL spectra of WO3, def-WO3and Cu0.029-def-WO3. 4c ). There were clearly six prominent characteristic signals of the DMPO-OOH adduct at hyperfine splitting constants of A N = 15.4 G and A H = 10.6 G over WO 3 , def-WO 3 and Cu 0.029 -def-WO 3 photocatalysts [66] . Cu 0.029 -def-WO 3 and def-WO 3 show 2.0 and 1.8 times stronger ·OOH production than the pristine WO 3 , due to the highly suppressed charge recombination induced by the cooperation of Cu single atoms and Ov. 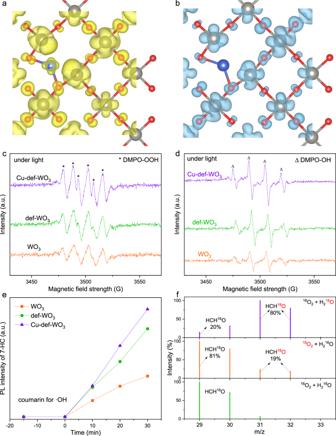Fig. 4: Photo-chemical properties. aConduction band minimum andbValence band maximum charge distributions of Cu-def-WO3. The grey, red and blue balls represent W, O and Cu atoms, respectively. In situ EPR monitor ofc·OOH andd·OH radicals trapped by DMPO over WO3, def-WO3and Cu0.029-def-WO3under light.eTime-dependent PL intensity of 7-hydroxycoumain from the reaction of coumarin and ·OH over WO3, def-WO3and Cu0.029-def-WO3.fGC-MS of the produced HCHO with isotopic labelled H218O or18O2in the presence of 19 bar CH4and 1 bar O2and 3 mL H2O over Cu0.029-def-WO3. 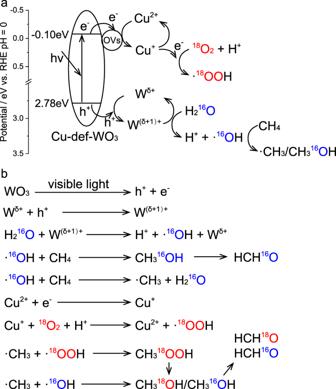Fig. 5: Proposed mechanism. a,bSchematic of charge transfer steps during selective CH4oxidation over Cu0.029-def-WO3. Figure 4d shows the four signal peaks (1: 2: 2: 1) of ·OH over the three photocatalysts. The trend of ·OH production from H 2 O oxidation with photo-induced holes (H 2 O + h + → ·OH + H + ) is similar to ·OOH production among WO 3 , def-WO 3 and Cu 0.029 -def-WO 3 , due to the enhanced charge separation. Quantification experiments further support that the production of ·OH radicals is directly associated with charge separation. The ·OH test using coumarin as the probe molecule (Fig. 4e ) supports that the Cu 0.029 -def-WO 3 is more efficient than the WO 3 and the def-WO 3 . Compared with the pristine WO 3 , the generation of the trapped species (coumarin + ·OH → 7-hydroxycoumain) is improved by 2.2 and 2.6 times for def-WO 3 and Cu 0.029 -def-WO 3 over a 30 min reaction, confirming improved ·OH radicals due to the synergy between Cu single atoms and Ov. Such trend is consistent with the in situ EPR under light. As ·OH could activate CH 4 to produce methyl radical (·CH 3 ) (·OH + CH 4 → ·CH 3 + H 2 O), a higher amount of ·OH produced would be more beneficial to CH 4 activation. Accordingly, both ·OOH and ·OH radicals are the reactive oxygen species during the photocatalytic CH 4 conversion. Initially, individual reactant adsorption was also simulated on the optimised photocatalysts. For oxygen adsorption on the Cu-def-WO 3 , simulation results reveal that the O 2 bond length is largely stretched to 1.41 Å in the molecular form on the Cu (Fig. S25 ). Due to the low oxidation states of the Cu δ+ , this stretched O 2 is further readily protonated to ·OOH. Further, water adsorption on the W δ+ site near an oxygen vacancy was compared on the optimised Cu-def-WO 3 and the pristine WO 3 surface (Fig. S26 ). The calculated free reaction energy is −0.78 eV and −0.65 eV, respectively, which indicates that both Cu and W δ+ enhance the interaction with water. The W δ+ with lower oxidation states ( δ < 6) near the O v defect is ready to host the lone-pair electrons from the water. Thus, both water and W δ+ present near the O v is the key to providing hole attraction and reaction sites for CH 4 activation. Since CH 4 could competitively react on the electron trapping site (Cu) or the hole trapping site (W δ+ ), the calculated free energy of the reaction is −0.04 and −0.43 eV on these two sites, respectively, as shown in the optimised geometries (Fig. S27 ), which indicates W δ+ site is the active site for methane activation. Nevertheless, it is still more difficult for CH 4 to be activated on W δ+ compared with H 2 O due to the much smaller free reaction energy of water (−0.78 eV), which then indicates CH 4 would be more likely to be directly activated by the ·OH radicals, rather than the photo-holes, through H 2 O oxidation with the photo-holes (Figs. S28 and S29 ). Oxygen sources of HCHO were further investigated through the isotopic experiment with 18 O 2 and H 2 18 O, separately. To confirm O 2 as the oxygen source, 1 bar 18 O 2 and 19 bar CH 4 over 20 mg Cu 0.029 -def-WO 3 with 3 mL H 2 O were utilised for a 6-h reaction. GC-MS results (Fig. 4f ) clearly show that the detected HCHO is composed of 81% HCH 16 O and 19% HCH 18 O, suggesting both O 2 and H 2 O are the oxygen sources for HCHO production. Meanwhile, a much higher content of HCH 16 O suggests H 2 O serves as the major oxygen source. Photocatalytic CH 4 conversion in the presence of isotopic labelled H 2 18 O further supports the primary role of H 2 O on HCHO production due to the reversed composition of 20% HCH 16 O and 80% HCH 18 O. The participation of H 2 O in HCHO formation suggests that the ·OH radicals formed from the oxidation of H 2 O with photo-induced holes (H 2 O + h + → ·OH + H + ) could directly react with CH 4 or ·CH 3 to form * CH 3 OH (“ * ” indicates it’s still adsorbed), and then to HCHO. Isotopic experiments were also conducted with 5 bar 13 CH 4 and 1 bar O 2 over 20 mg Cu 0.029 -def-WO 3 in 3 mL H 2 O for a 6-h reaction. 13 C nuclear magnetic resonance (NMR) spectroscopy in Fig. S30 shows only one signal at 82.2 ppm, assigned to HO 13 CH 2 OH, which was the diol structure of H 13 CHO in an aqueous solution (H 13 CHO + H 2 O → HO 13 CH 2 OH) [18] , [20] . This result confirms that the carbon source of the produced HCHO comes from CH 4 . Moreover, it also confirms the high selectivity with no CH 3 OH and HCOOH production, consistent with the 1 H NMR results (Fig. S31 ). Based on the above results, particularly based on the strong evidence of the characteristics of the ·OH and ·OOH radicals by in situ EPR, a radical mechanism (Fig. 5a, b ) of aerobic photocatalytic CH 4 conversion to HCHO is proposed here over the Cu 0.029 -def-WO 3 catalyst, which consists of nanocrystalline WO 3 substrate with single atoms Cu δ+ and O v /(W δ+ ). In general, under visible-light irradiation, electrons are excited from the valence band (VB) to the conduction band (CB) of WO 3 . The active electrons then migrate to Cu 2+ to form Cu + (Cu 2+ -e - ). The adsorbed O 2 on the Cu site next reacts with the electrons trapped by Cu + to form the ·OOH radical, which requires a potential of −0.046 eV [63]. In parallel, photo-induced holes are trapped by the W δ+ with low oxidation (W δ+ + h + → W (δ+1)+ ), and then react with the chemical adsorbed H 2 O at the oxygen vacancy induced W δ+ site to form ·OH radicals. Meanwhile, the ·OH radical could directly activate CH 4 and then react with ·CH 3 to form * CH 3 OH intermediate, then being transformed to the desired HCHO. The absence of CH 3 OOH and CH 3 OH in 1 H NMR spectra (Fig. S32 ) may be attributed to the immediate conversion of such intermediates to HCHO. On the basis of efficient activation of the different reactants (H 2 O, O 2 and CH 4 ) with the assistance of the specific synergy of O v induced W δ+ site and highly dispersed Cu atomic co-catalyst, the selectivity of HCHO over Cu 0.029 -def-WO 3 was successfully maintained at nearly 100% over a long period of time to 10 h. Fig. 5: Proposed mechanism. a , b Schematic of charge transfer steps during selective CH 4 oxidation over Cu 0.029 -def-WO 3 . Full size image In summary, an effective strategy to overcome the dilemma of enhancing the efficient activation while suppressing the over-oxidation of CH 4 has been developed for the selective production of value-added HCHO over a noble-metal-free Cu 0.029 -def-WO 3 photocatalyst. The WO 3 substrate provides the visible-light responsive activity for CH 4 conversion, while the atomically dispersed Cu acts as an effective electron acceptor, as indicated from the analysis of the in situ XPS and EPR spectra under light irradiation. O v induce the formation of reactive W δ+ species, which further enhances the selective chemical adsorption and activation of H 2 O. The coordinated ensemble of the dual active sites synergistically leads to efficient charge separation and transfer. As a result, under visible-light irradiation at room temperature, a superior photocatalytic CH 4 conversion efficiency has been achieved with a high TOF of 8.5 × 10 6 μmol (HCHO) ·g −1 (cocatalyst) ·h −1 , out-performing previously reported photocatalysts, even much better than the noble-metal photocatalytic processes [19] . Nearly 100% selectivity and a high HCHO evolution rate of 4979.0 μmol·g −1 have been achieved under 420 nm light irradiation at room temperature. Isotopic experiments provide strong evidence that both O 2 and H 2 O are the oxygen sources for HCHO production, with H 2 O being the major one. This work provides a new avenue for simultaneous regulation of CH 4 activation under visible-light irradiation and suppression of over-oxidation by incorporation of adjacent dual active sites, which is of great interest in net-zero green conversion and upgrading of natural resources to high-value chemicals. Preparation of Cu x -def-WO 3 Cu x -def-WO 3 photocatalysts were prepared by a highly reproducible incipient impregnation method and subsequent hydrogen reduction. In a typical experiment, 5.0 g WO 3 was first mixed with 2.0 mL CuCl 2 aqueous solution containing a certain amount of CuCl 2 . After uniformly stirring and ageing at ambient temperature overnight, the obtained solid was dried at 60 o C for another 12 h. The dried samples were then grounded and calcined at 250 o C for 2 h at a ramping rate of 5 o C/min in 5 vol.% H 2 /Ar flow (80 mL/min). The as-prepared samples were denoted Cu x -def-WO 3 , where x % represented the mass percentage of the copper atom. For comparison, the defective WO 3– x (denoted def-WO 3 ) was prepared under identical conditions but without CuCl 2 addition. Characterisations XRD patterns were acquired on the D8 ADVANCE diffractometer ( Bruker Co., Ltd ). Raman spectra were acquired on the DXR 2DXR2 instrument ( Thermo Fisher Scientific, Co., Ltd ). XPS spectra were measured with the PHI 5000 Versa Probe III instrument ( ULVAC-PHI Co., Ltd ). In situ XPS spectra were collected in dark or under visible-light irradiation for 20 min on the Thermo ESCALAB 250Xi instrument with an Al Kα radiation source. In situ solid-state EPR spectra were measured on the ELEXSYS II EPR instrument with 20 mg photocatalyst in dark or under 420 nm light irradiation. HRTEM images were captured on the Talos F200X instrument ( FEI Co., Ltd ). Where photocatalyst was pre-dispersed under sonication and dipped on the molybdenum mesh as the copper-free supporting substrate. UV–vis DRS spectra were recorded on the UV-3600 Plus spectrometer ( Shimadzu Co., Ltd ) with spectroscopic pure BaSO 4 as the references. Steady-state and time-decay PL spectra were recorded at room temperature on the QM400 and FLSP920 spectrofluorometers, respectively. Photocatalytic methane conversion Photocatalytic CH 4 conversion reaction was conducted in the 200 mL stainless-steel high-pressure reactor equipped with Teflon lining. Typically, 5 mg photocatalyst was first dispersed in 120 mL distilled H 2 O under stirring. The reactor was then sealed and purged with ultrapure oxygen (99.99 vol.%) under moderate stirring for about 20 min to remove the air completely. After acquiring atmospheric oxygen or desired partial pressure, ultrapure CH 4 (99.99 vol.%) was injected into the reactor to achieve total pressure of 20 bar. The reactor with top-irradiation was then irradiated with the LED lamp source (420 nm, PLS-LED100C , Beijing Perfectlight Technology Co., Ltd ). Photocatalytic reaction was conducted for 2 h at 25 o C. The gaseous products were measured by gas chromatograph ( GC2014 , Shimadzu Co., Ltd ) equipped with a thermal conductivity detector and flame ionisation detector. The dissolved CO 2 was also analysed through the precipitation method with excessive Ba(OH) 2 , where excess Ba(OH) 2 was added into 10 mL supernate after reaction [67] . No discernible precipitation was observed, indicating the dissolved CO 2 was too low to be measured. The possible existence of other products, including CH 3 OOH, CH 3 OH and HCOOH, was analysed by 1 H nuclear magnetic resonance spectroscopy ( AVANCE III, JEOL Ltd ). The results (Fig. S31 ) confirmed that no CH 3 OOH, CH 3 OH and HCOOH were produced during the CH 4 conversion reaction by the photocatalyst. HCHO was measured by the colorimetric method based on the reaction between acetylacetone and HCHO in the presence of acetic acid and ammonium acetate [68] . A trace amount of CO 2 was detected during all photocatalytic reactions, demonstrating the ultrahigh HCHO selectivity. Reusability of Cu 0.029 -def-WO 3 was tested by photocatalytic CH 4 conversion. Parallel experiments was conducted under identical conditions to replenish the losses of photocatalyst. After each experiment, the reactant was centrifuged and dried at 60 o C in vacuum. Then 5 mg collected photocatalyst was re-used for the next cycling experiment. Isotopic experiments For carbon source investigation with isotopic labelled 13 CH 4 : 20 mg Cu 0.029 -def-WO 3 photocatalyst was dispersed in 3 mL H 2 O, then the reactor was vacuumed for 30 min and refilled with 1 bar O 2 and 5 bar 13 CH 4 . The reaction was conducted for 6 h to gain more concentrated products for detection facilitation. As H 13 CHO tended to exist as HO 13 CH 2 OH in aqueous solution, the products were identified by 13 C NMR ( AVANCE III , JEOL Ltd ). For oxygen source investigation with isotopically labelled 18 O 2 : 20 mg Cu 0.029 -def-WO 3 photocatalyst was dispersed in 3 mL H 2 O, then the reactor was vacuumed for 30 min and refilled with 1 bar 18 O 2 and 19 bar CH 4 . The reaction was conducted for 6 h to gain more concentrated products for detection facilitation. The as-produced HCH 18 O was measured with GC-MS ( QP2020, Shimadzu Co., Ltd ) equipped with the Cap WAX column to identify the existence of H 2 18 O. For oxygen source investigation with isotopic labelled H 2 18 O: 20 mg Cu 0.029 -def-WO 3 photocatalyst was dispersed in 3 mL H 2 O, then the reactor was vacuumed for 30 min and refilled with 1 bar 18 O 2 and 19 bar CH 4 . The reaction was conducted for 6 h to gain more concentrated products for detection facilitation. The as-produced HCH 18 O was measured with GC-MS ( QP2020, Shimadzu Co., Ltd ) equipped with the Cap WAX column to identify the existence of H 2 18 O. Photoelectrochemical measurements Mott-Schottky plots, electrochemical impedance spectroscopy (EIS) and photocurrent density were measured on the three-electrode system with an electronic workstation ( CHI660E ). Photocatalyst coated by indium tin oxide (ITO) glass (10 × 10 mm), Ag/AgCl electrode and platinum sheet electrode were respectively employed for working, reference and counter electrodes, with 0.1 mol·L −1 Na 2 SO 4 solution as the electrolyte. The working electrodes were prepared by scraping the paste-like mixture containing 100 mg of different photocatalysts, 450 μL ethanol and 50 μL Nafion solution ( Shanghai Adamas Reagent Co., Ltd ). Before measurement, the working electrodes were dried at 60 °C in vacuum. Monitor of the reactive oxygen species 5, 5-dimethyl-1-pyrroline N-oxide (DMPO) was used as the trapping agent for the monitoring of the reactive oxygen species, including hydroperoxyl (·OOH) and hydroxyl (·OH) radicals. For monitoring the generation of ·OOH radical, 10 mg Cu 0.029 -def-WO 3 photocatalyst was dispersed in 5 mL methanol in the dark and purged with ultrapure O 2 (99.99 vol.%) for 20 min. For monitoring the generation of ·OH radical, 5 mg Cu 0.029 -def-WO 3 photocatalyst was dispersed in 5 mL distilled H 2 O in the dark and purged with ultrapure argon (99.99 vol.%) for 20 min. In situ EPR spectra of the above suspension in dark and under light were then obtained on the ELEXSYS II EPR instrument. Analysis the productivity of ·OH radical Coumarin was used as the probe to evaluate the productivity of ·OH radical due to the reaction between coumarin and ·OH to produce 7-hydroxycoumain (7HC). Typically, 20 mg Cu 0.029 -def-WO 3 photocatalyst was dispersed in 100 mL aqueous coumarin solution (0.5 mM). After stirring in dark for 30 min, 5 mL reactant was sampled every 5 min under 420 nm light irradiation. After filtration, the PL spectra of the formed 7HC were measured by F4500 spectrofluorometer. Theoretical calculations All the calculations were performed based on density functional theory (DFT), implemented in the Vienna ab initio Package (VASP) [69] . Electron-ion interactions were described with the projector-augmented-wave (PAW) method with an energy cut-off set to 500 eV [70] . The PBE functional was used to optimise the structural models and to analyse the electronic structures [71] . The structures were fully relaxed until the changes in energy and in the force upon ionic displacement were no greater than 10 −5 eV and 0.02 eV/Å, respectively. The delocalised electron was treated by the (DFT + U) Dudarev approach with the effective U value set to 5 and 8 for tungsten and copper, respectively [72] . The U values are in line with previous calculations on WO 3 [73] . Due to the complex oxidation states of Cu in Cu-def-WO 3 , we have adopted the U value from one report [74] , as this U value has been well assessed for Cu 2 O, CuO and Cu 3 O 4 . The partial charges were determined using the Bader charge analysis [75] . The chemical potential of Cu single atom is derived from the bulk copper. The entropy of gas phase H 2 O, O 2 , HCHO are obtained from the NIST database under standard conditions [76] . The adsorption energy ( E ad ) is calculated by 
    E_ad=E_total-E_adsorbent-E_sub
 (2) where the E total , E adsorbent and E sub is the total energy of the system, the energy of the adsorbent and the substrate, respectively. The reaction free energy is calculated according the following equation: 
    G=E_ad+ZPE-T S
 (3) where the E ad is the adsorption energy, ΔZPE is the changes of the zero point energy, Δ S is the changes of the entropy of the reaction. The internal thermal energy U 0→ T is calculated based on 
    U_0→ T=RT^2(δlnq/δ T)_V
 (4) The reaction temperature is set to 300 K.